Cryo-EM structure of mycobacterial cytochromebdreveals two oxygen access channels Cytochromes bd are ubiquitous amongst prokaryotes including many human-pathogenic bacteria. Such complexes are targets for the development of antimicrobial drugs. However, an understanding of the relationship between the structure and functional mechanisms of these oxidases is incomplete. Here, we have determined the 2.8 Å structure of Mycobacterium smegmatis cytochrome bd by single-particle cryo-electron microscopy. This bd oxidase consists of two subunits CydA and CydB, that adopt a pseudo two-fold symmetrical arrangement. The structural topology of its Q-loop domain, whose function is to bind the substrate, quinol, is significantly different compared to the C-terminal region reported for cytochromes bd from Geobacillus thermodenitrificans ( G. th ) and Escherichia coli ( E. coli ). In addition, we have identified two potential oxygen access channels in the structure and shown that similar tunnels also exist in G. th and E. coli cytochromes bd . This study provides insights to develop a framework for the rational design of antituberculosis compounds that block the oxygen access channels of this oxidase. Respiratory oxygen reductases (terminal oxidases) comprise a series of structurally distinct enzymes that are widely distributed across all kingdoms of life. The heme-copper oxidases (HCO) and bd -type oxidases (cytochromes bd ) are two well-known types of membrane-integrated terminal oxidases [1] , [2] . They catalyze the reduction of molecular oxygen (O 2 ) to water by the respiratory substrate, cytochrome c or quinol, coupled to the generation of a proton motive force utilized for adenosine triphosphate (ATP) synthesis [3] , [4] . Compared to the well-characterized HCOs, cytochromes bd have not been widely studied. These cytochromes are only present in prokaryotes, which include many human pathogens, and thus belong to an evolutionarily distinct oxidase family [4] . Cytochrome bd oxidases possess a high affinity for oxygen [5] , [6] , which facilitates bacterial survival under O 2 -poor environments [7] , [8] . Apart from this, cytochromes bd also endow bacteria with a number of vitally important physiological functions including enhancing tolerance to nitrosative stress [9] , contribute to resistance to hydrogen peroxide [10] , suppress extracellular superoxide production [11] , and confer the ability to defend against antibacterial agents [12] . It is likely that these properties of cytochromes bd promote virulence in a number of bacterial pathogens that cause serious infectious diseases to humans, such as Mycobacterium tuberculosis [13] , Brucella abortus [14] , as well as Salmonella Typhimurium [15] , [16] , Bacteroides [7] , and Listeria monocytogenes [17] . Since cytochrome bd is a key enzyme for the survival of prokaryotes and is absent in mammals, it is a promising therapeutic target for the development of antibacterial agents [4] , [18] . To date, two structures of the bd oxidases have been reported. One is from Geobacillus thermodenitrificans ( G. th ) [19] and the other is from Escherichia coli ( E. coli ) [20] , [21] . These enzymes possess two key subunits CydA and CydB but vary in the numbers of additional small subunits that are associated with them. G. th bd oxidase contains an association subunit called CydS and E. coli bd oxidase includes two association subunits named CydX and CydH (or CydY). Common features in these complexes are two b -type hemes (low-spin heme b 558 and high-spin heme b 595 ) and one d -type heme which are arranged in a triangular manner but with different relative positions in the two structures. These observations suggest that homologous bd oxidases share a similar architecture but can vary in mechanistic detail [21] , [22] , [23] , [24] . Therefore, more structural information is needed to obtain a comprehensive knowledge of the structure and function of bd oxidases. The properties of several mycobacterial cytochromes bd have been investigated [12] , [18] , [24] , [25] , but given they share only a low sequence identity (the lowest similarity score is 20%) with the two previously reported cytochrome bd structures it is difficult to rationalize the function of these cytochromes bd [18] . In the present study, we have determined a 2.8 Å cryo-electron microscopy (cryo-EM) structure of a dimeric bd oxidase from Mycobacterium smegmatis ( Msm ). In so doing, we have identified two potential oxygen access channels, which could be excellent targets for anti-tuberculosis drug discovery. Overall structure of Mycobacterium smegmatis bd oxidase Msm bd oxidase was recombinantly expressed and purified to homogeneity (Supplementary Fig. 1a–d ). The purified Msm bd enzyme is a stable and functional assembly with a turnover number of 21.6 ± 2.8 e − s −1 (Supplementary Fig. 1e ). A 2.8 Å resolution structure was determined in lipid nanodiscs using cryo-EM. Details for data collection and model statistics are provided (Supplementary Fig. 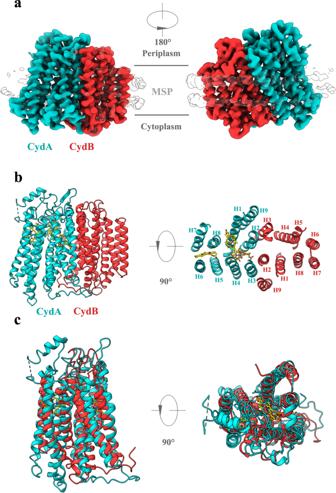Fig. 1: Overall structure of theMsm bdoxidase. aThebdoxidase cryo-EM density map at 2.8 Å resolution. MSP, membrane scaffold protein.bCartoon representation of thebdoxidase consisting of subunits CydA (red) and CydB (cyan).cStructural superposition of CydA and CydB. 2 and Supplementary Table 1 ). Although the construct design, expression, and purification of Msm bd oxidase were performed according to a procedure described previously for G. th [19] and E. coli [20] , [21] bd oxidases, only CydA and CydB were observed. No additional small subunit similar to CydS/X or CydH/Y found in the G. th [19] and E. coli [20] , [21] bd oxidases were observed in the Msm complex, noting that in the G. th and E. coli studies, the genes coding for the associated subunits CydS/X of G. th [19] bd oxidase and CydH/Y of E. coli [20] , [21] bd oxidase were not included in the corresponding expression plasmid. Nonetheless, these two small subunits were observed to co-elute upon purification in both complexes. Thus, we believe that the Msm bd oxidase contains only two core subunits, CydA and CydB (Fig. 1a, b, and Supplementary Figs. 3 , 4 ). This hypothesis is further supported by a BLAST search of the mycobacterial genomes which did not identify any subunits homologous to CydS/X and CydH/Y (Supplementary Fig. 5 ). In addition, Msm bd oxidase in the absence of associated subunits is active, whereas the E. coli bd oxidase is not active in the absence of its associated subunits [26] . In summary, mycobacterial bd oxidase appears to only consist of the two core subunits and no other units. Notably, there is a high structural similarity between the G. th and E. coli counterparts compared to Msm core subunits, except for a little difference in the topology of CydB subunits between Msm and E. coli (Supplementary Fig. 6 ). Fig. 1: Overall structure of the Msm bd oxidase. a The bd oxidase cryo-EM density map at 2.8 Å resolution. MSP, membrane scaffold protein. b Cartoon representation of the bd oxidase consisting of subunits CydA (red) and CydB (cyan). c Structural superposition of CydA and CydB. Full size image In terms of secondary structure, Msm bd oxidase, CydA, and CydB possess a common fold each consisting of nine transmembrane helices (TMHs). These two subunits are related by an approximate two-fold rotational axis of symmetry. The TMH domains can be divided into two four-helix bundles and one additional peripheral helix (Fig. 1c ). The domains of the two subunits superpose well with a root mean square deviation of 3.6 Å for all the Ca atoms (Fig. 1c ) and thus suggest that CydA and CydB evolved by a gene duplication event. The three heme groups ( b 558 , b 595 , and d ) are clearly visible in the CydA subunit (Fig. 1b and Supplementary Fig. 3 ). Given the two other bd oxidases have associated subunits in their structures, our structure suggests that their presence is species-dependent. Q-loop of M. smegmatis bd oxidase The bd oxidases are divided into the S (short)- and the L (long)-subfamilies [4] . This is according to the length of the region of polypeptide referred to as the Q-loop (quinol-binding domain). Mycobacterial cytochromes bd belong to the S-subfamily [20] . The Q-loop of CydA has a water-exposed domain (segment 257–339), connecting the 6 and 7 in the hydrophilic extracellular space [19] , [20] , [21] . It has two parts, one associated with the N-terminal domain (Q N ) and the other with the C-terminal domain (Q C ). The Q N -loop plays a functional role in the binding and oxidation of the quinol [27] , [28] and the Q C -loop is needed for the assembly/stability of the enzyme [22] , [23] , [25] . In the present study, the densities corresponding to the Q-loop without and with aurachin D (a quinone analog inhibiting mycobacterial cytochrome bd ) bound are not completely resolved (Supplementary Figs. 2 and 7 ). A comparison of these two structures does not show any conformational changes which may be a function of the resolution of the data or the fact that the region around the aurachin D is inherently disordered. Aurachin D is bound to the Q N -loop [20] , potentially stabilizing the Q-loop, and has the ability to inhibit the activity of Msm cytochrome bd [29] . The structure of the Q N -loop in the E. coli enzyme is also not fully resolved [20] , [21] . Therefore, these structural data suggest that the Q N -loop is intrinsically flexible. Its flexibility may be required for the rapid binding and release of the quinols. The remaining segments of the Q-loop in the Msm bd oxidase structure are well resolved. At the periplasmic side of TMH 6, there is a short horizontal helix, Q h1 , that includes the highly conserved residues Lys 260 and Glu 265 (Lys 252 and Glu 257 in G. th and E. coli ) [19] , [20] , [21] , critical for quinol substrate binding and electron transfer [28] (Fig. 2a ). The structure of Qh1 is conserved with respect to the G. th and E. coli enzymes [19] , [20] , [21] (Fig. 2b ). It is noteworthy that the Q C -loop here adopts a rigid secondary structure with a horizontal Q h2 (residues 317–327), that emerges from the flexible Q N -loop part and covers the periplasmic surface of CydA. Site-directed mutagenesis and whole-bacteria assays, performed on the Mycobacterium tuberculosis ( Mtb ) bd oxidase, demonstrated that the regions corresponding to the Q h2 and the equivalent residues Tyr 323 , Phe 327, and Tyr 332 nearby the Q h2 stretch are essential for the function of the oxidase [25] (Supplementary Fig. 8 ). In Msm bd oxidase, we observe that these three residues are involved in the interactions with Q h1 and the periplasmic loop between TMH 8/9, located at the periplasmic surface of heme groups b 558 and b 595 , and as a result potentially affect the cofactor and quinol binding (Fig. 2a ). Tyr 323 forms the van der Waals interaction with Pro 258 in the Qh1 region, and Phe 327 and Tyr 332 form the stacking interactions with Trp 404 in the loop TM8/9 region. So the observed structural features are in agreement with the previous functional characterization of the Mtb enzyme [25] . Additionally, according to the structural superposition between Msm and E. coli CydA subunits (Supplementary Fig. 6 ), the corresponding residues of Tyr 323 , Phe 327 , and Tyr 332 in Msm are His 314 , Tyr 353 , Ser 379 in E. coli , respectively. His 314 and Tyr 353 also form van der Waals interactions and a stacking interaction, respectively, with Thr 251 in the Qh1 region and Trp 451 in the loop TM8/9 region. Hence, these interactions in the Msm bd oxidase are very similar to those observed in the E. coli complex. It is also worth noting that the folding of the Q C -loop region is different (Fig. 2b ), compared to the other bd oxidases, though the Q-loop domain of Msm bd oxidase should be remembered these belong to the short Q-loop class (Supplementary Fig. 9 ) [20] . This array of differences suggests that the Q-loop domain could be used as a marker for evolutionary analysis of bd oxidases in prokaryotes (Supplementary Fig. 10 ). Fig. 2: The Q-loop in bd oxidases. In CydA, a hydrophilic region between the transmembrane helices 6 and 7 harbors the quinol-binding site and has thus been named the Q-loop. a The N-terminal and C-terminal Q loops are rigid and well-ordered helical segments, but the linking region between them is not resolved in the maps. The residues labeled are important for stability or activity. b The bd oxidases from G. th , E. coli , and Msm are superimposed. The Q-loop domains from G. th , E. coli , and Msm are shown in red, blue, and cyan, respectively. Full size image Electron transfer in Msm bd oxidase The three heme groups ( b 558 , b 595 , and d ) unambiguously identified in Msm bd oxidase are organized in a triangulated arrangement near the periplasmic side of CydA (Fig. 3a ). In this structure, the low-spin b 558 is within the transmembrane core of subunit CydA, adjacent to the Q N -loop segment. Its axial ligands are conserved residues His 185 and Met 346 (His 186 and Met 325 in G. th ; His 186 and Met 393 in E. coli ) [19] , [20] , [21] (Fig. 3b ). Heme b 595 is located closer to the periplasmic side and is ligated by Glu 398 (Glu 378 in G. th ; Glu 445 in E. coli ) [19] , [20] , [21] (Fig. 3b ). There is a conserved Trp 394A between heme groups b 595 and b 558 that may mediate electron transfer [19] , [20] , [21] , [30] . The third cofactor heme d , the site of oxygen binding and reduction, is positioned at the center of CydA and the invariant His [18] (His [21] in G. th ; His [19] in E. coli ) appears to be ligated to the heme iron on one side [19] , [20] , [21] . Fig. 3: Cofactor organization in Msm cytochrome bd . a Triangular arrangement of the heme cofactors in CydA. Heme edge-to-edge distances are indicated by numbers in the parentheses. b Axial amino acid ligands of the heme cofactors. c Heme superposition between E. coli , G. th , and Msm . d The superimposed heme d sites from Msm and E. coli . Full size image Although the bd oxidases of G. th and Msm are from the same S-subfamily, the relative arrangement of the three heme groups are strikingly different [19] (Fig. 3c ). The organization of the redox center in Msm cytochrome bd is similar to that reported for the L-subfamily as exemplified by E. coli bd oxidase [20] , [21] . A structural superimposition (Fig. 3c ) shows the two heme groups are located in the same position in the CydA, the distances between the central iron atoms are consistent as the orientations of the heme planes relative to the membrane plane. Therefore, the cofactor location is a conserved feature of the three respiratory bd oxidases. On the opposite side of the heme d , Glu 98 (Glu 101 in G. th ; Glu 99 in E. coli ) acts as the axial ligand. Glu 98 here is 6.2 Å from the central iron atom. The equivalent distances in G. th and E. coli are 2.1 and 6.0 Å, respectively [19] , [20] , [21] . This voluminous cavity is suggested to be used for the binding of substrates such as oxygen, roofed by the hydrophobic Ile 143 and Phe 103 (Ile 144 and Phe 104 in E.coli ) [20] , [21] . The location and surrounding environment of the cofactors in the bd oxidase are highly conserved between Msm and E. coli (Fig. 3d ). Collectively, it is suggested that a sequential electron transfer from heme b 558 via heme b 595 to heme d also exists in the mycobacterial bd oxidases [20] , [21] . Two oxygen access channels in Msm bd oxidase Cytochromes bd play a role in energy metabolism with high O 2 affinity under hypoxic conditions [4] , [12] , conditions often encountered by the microorganisms in their natural habitats. The dioxygen has to bind to heme d and then is reduced at this position [19] , [20] , [21] . In E. coli bd oxidase, the O 2 -channel acts as a pathway for direct oxygen diffusion from the membrane interior to the heme d reaction site. It is formed by a small direct hydrophobic channel, which starts above Trp 63 (Trp 67 in Msm ) at the membrane interface between TMH1 and TMH9 of CydB and extends further to heme d on CydA [20] , [21] . The corresponding residue Trp has been demonstrated to be essential for bd activity in Mtb [25] . Noteworthy, in the Msm structure, the channel is also formed by a conserved structural topology and residues according to a comparison between the bd oxidases from E. coli and Msm (Supplementary Fig. 11 ), which suggests that the oxygen here may also access the active site through this conserved O 2 -channel (identified as channel 1) (Fig. 4 ). Intriguingly, there is an additional accessible channel directly connecting to the protein surface and extending to the heme b 595 , which is also identified in the G. th enzyme [19] . This channel has also been proposed for the oxygen entry site in G. the bd oxidase [19] , [20] , which is blocked by the single-transmembrane subunit CydH in the E. coli enzyme [20] , [21] . In addition, the heme d in this structure is buried deeper inside the subunit CydA and the penetration of dioxygen from this cavity into heme d is also blocked by heme d itself [21] . However, the channel is accessible in the Msm enzyme and previous studies have reported that the high-spin heme b 595 could be the second reaction site for O 2 [5] , [31] . Therefore, this channel (channel 2) is very likely to be an alternative pathway to guide dioxygen to heme b 595 , which may further sustain energy metabolism in the bacterial cell and enhance mycobacterial survivability in the host. It has been reported that the threshold pO 2 (O 2 tension) of the growth medium for the induction of cyd gene cluster in M. smegmatis (ca. 1% air saturation) [32] is significantly lower than that of E. coli (10% air saturation) [33] , suggesting that the Msm bd oxidase has a different functional or kinetic range with respect to oxygen availability compared to that of E. coli [32] . Overall, therefore, the two oxygen channels in Msm bd oxidase are reasonably proposed based on these structural features and the previously described studies. Future investigations are needed to determine whether these two catalytic reactions take place at the same time. Fig. 4: Proton/gaseous substrate channels in the Msm bd oxidase. Subunits CydA/B are shown in cartoon representation. The putative dioxygen and proton channels are labeled. The heme groups are shown as stick models. The proton transfer step from heme b 595 to heme d is identified by a black dashed path. Full size image Although the bd oxidases do not pump protons from the cytoplasmic side to periplasmic side, producing the proton motive force across the membrane, the pathway for proton uptake from the cytoplasm is crucial to reduce dioxygen to water [4] . Two proton pathways in subunits CydA and CydB from the cytoplasmic side to the active site have been proposed in G. th [19] and E. coli enzymes [20] , [21] . These studies indicate two hydrophilic channels for proton transfer. Based on the superimposition and structural analysis between the bd oxidases from G. th and E. coli [19] , [20] , the relatively conserved hydrophilic residues in our model, along the canonical CydA and CydB pathways, are His 125.A , Gln 36.A , Glu 106.A , Ser 107.A , Ser 139.A to Glu 98.A , and Asp 25.B , Asp 62.B , and Asn 64.B (Fig. 4 , Supplementary Fig. 11 ). Given the conserved identity of the proton pathways in mycobacterial enzymes, they are also likely to facilitate proton transfer for dioxygen reduction at the heme d site. In addition, in terms of the dioxygen reduction at the heme b 595 site, there must be an additional proton transfer step from heme d to heme b 595 in order to deliver protons to the oxygen reduction site (Fig. 4 ), which may be potentially similar to that of the G. th enzyme [19] . According to the current structure, the heme propionate of heme d is in a hydrophobic environment without any charge compensation. It is thus very likely protonated and supplies protons for unresolved water molecules here that connect heme b 595 to heme d . These protons would be replenished via the CydA/B proton pathways. Overall, the electron released from the quinol bound at the quinone-binding site is transferred, in turn, to the prosthetic groups heme b 585, heme b 595 to heme d . At the same time, the oxygen molecule that is diffused to the heme b 595 and/or heme d sites is reduced to water, a process that is involved in conducting protons to the oxygen-binding site through the CydA/B pathways (Fig. 5 ). Fig. 5: A schematic diagram showing the electron/proton transfer pathway in Msm bd oxidase and the relevant oxygen entry pathway. The heme groups are shown as in stick models. The putative dioxygen and proton channels are labeled. Electron transfer directions are shown in black arrows. Full size image Cytochromes bd is ubiquitous among prokaryotes (but not present in eukaryotes) and is now attracting attention as promising targets for next-generation antibacterials. Here, we have determined the 2.8 Å cryo-EM structure of Msm bd oxidase. The overall fold is similar to the two other previously reported bd oxidases but exhibits several different features, including the fold of the Q-loop and the number of associated subunits. In addition, we have identified two potential oxygen access channels that look to be also present in G. th and E. coli cytochromes bd . The quinol-binding site located in the Q-loop has been proposed to be a target for drug discovery. However, the structure of the Q-loop has not been fully determined, thus posing a challenge for the design of quinol-type inhibitors. The two oxygen-conducting O 2 -channels could be alternative targets for the discovery of anti-tuberculosis drugs. Bacteria strain and culture The cydAB gene was cloned into pMV261 plasmid with a 10x His tag at the C-terminus of cydB . 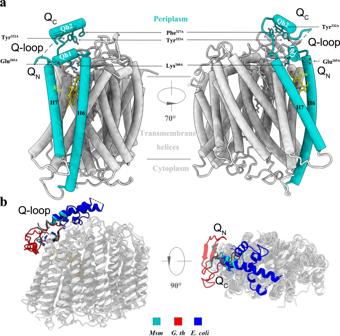Fig. 2: The Q-loop inbdoxidases. In CydA, a hydrophilic region between the transmembrane helices 6 and 7 harbors the quinol-binding site and has thus been named the Q-loop.aThe N-terminal and C-terminal Q loops are rigid and well-ordered helical segments, but the linking region between them is not resolved in the maps. The residues labeled are important for stability or activity.bThebdoxidases fromG. th,E. coli, andMsmare superimposed. The Q-loop domains fromG. th,E. coli, andMsmare shown in red, blue, and cyan, respectively. The primers are listed in Supplementary Table 2 . Expression was achieved by electroporation of the plasmid into strain Msm mc 2 51 [34] . A volume of 1 mL strain stock was added to 24 mL LB broth (0.1% Tw80, 50 μg/mL kanamycin, and 20 μg/mL carbenicillin) and cultured overnight at 37 °C and 220 rpm. Next, 4 mL pre-culture aliquots were transferred to 1 L LB broth (rubber plug, 0.1% Tw80, 50 μg/mL kanamycin, and 20 μg/mL carbenicillin) and cultured at 37 °C and 220 rpm. When the OD 600 reached 0.8, 5 mL of 40% acetamide was added to induce the expression of the target protein over 3 days at 25 °C and 220 rpm. Protein purification and characterization The purification procedure followed a previous study but with a few modifications [30] . Membranes of the cells were extracted in buffer (20 mM HEPES, pH 7.4, 100 mM NaCl), and then stirred slowly at 4 °C for 2 h with 1% (w/v) dodecyl-beta-d-maltoside (DDM). The supernatant after centrifugation was loaded onto a Ni-NTA column and the eluted fraction including the protein of interest was loaded onto a Superdex 200 (GE Healthcare) column equilibrated in a buffer containing 20 mM HEPES, pH 7.4, 100 mM NaCl, and 0.02% (w/v) DDM. The peak fractions were analyzed by SDS–PAGE (sodium dodecyl sulfate–polyacrylamide gel electrophoresis), then pooled and concentrated to 6 mg/mL. Preparation of reduced quinol substrate 2,3-Dimethyl-1,4-naphthoquinone (DMNQ, CAS 2197-57-1) was synthesized by WuXi AppTec. DMNQ reduction was performed following previously published protocols with some modifications [35] . To prepare the reduced quinol, DMNQH 2 , 20 mM DMNQ was ultrasonically dissolved in 1 mL ethanol with 6 mM HCl. A few grains of sodium borohydride (NaBH 4 ) were then added to obtain a fully reduced, colorless solution in the ice-bath. An appropriate amount of HCl was used to quench the mixture under the protection of argon. The quinol solution was stored at −80 °C. Oxygen consumption assay Oxidase activity was determined according to the previous studies [20] , [36] , [37] . Oxygen consumption was monitored with a Clark-type oxygen electrode (Hansatech Chlorolab 2) in the buffer 20 mM HEPES, pH 7.4, 100 mM NaCl, 0.04% DDM, and 10 mM DTT at room temperature. To begin the assay, 480 μL buffer was first added until the oxygen equilibrium. 20 μL DMNQH 2 was then added and the substrate autoxidation rate was recorded. The reaction was started by the addition of 0.8 μM bd complex. The time course for oxygen consumption was curved with GraphPad prime 6.0 software, from which an estimate of the observed pseudo-first-order rate constant ( k obs ) is obtained (corrected for autoxidation). This assay included four groups of parallel experiments. Reconstruction of cytochrome bd into nanodiscs MSP1D1 was used to reconstruct the nanodisc and the purification and reconstruction followed the reported study [38] . Briefly, cytochrome bd , MSPD1, and POPC were mixed with a stoichiometry of 1:4:160 and incubated at 4 °C for one hour. Next, 200 μL of resuspended Bio-Beads (0.5 g/mL) were added twice with an interval of 30 min to remove the detergents. After 12 h of incubation, the supernatant was applied to a Superdex 200 (GE Healthcare) column equilibrated in 20 mM HEPES, pH 7.4, 100 mM NaCl buffer. The peak fraction was collected and concentrated. Cryo-EM sample preparation and data collection Aliquots (4 μL) of reconstructed nanodisc-cytochrome bd at a concentration of 1 mg/mL were applied to glow-discharged Quantifol Cu 1.2/1.3 (mesh 300) grids. For cytochrome bd and aurachin D complex, 0.35 mM aurachin D was added and incubated with nanodisc-cytochrome bd for half an hour before sample vitrification. Glow discharge was accomplished by adding an H 2 and O 2 mixture in the Gatan Solarus 950 for 25 s. After blotting for 3 s with a blot force of −2, grids were flash-frozen in liquid ethane cooled by liquid nitrogen using an FEI Vitrobot operated at 8 °C and 100% humidity. For cytochome bd complex without aurachin D, data collection was achieved using the Titan Krios electron microscopy operated at 300 kV with a Gatan K3 detector at a magnification of SA ×29,000. Images were recorded in super-resolution mode binned to a pixel size of 0.82 Å/pixel. 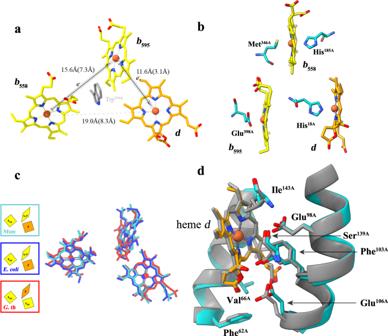Fig. 3: Cofactor organization inMsmcytochromebd. aTriangular arrangement of the heme cofactors in CydA. Heme edge-to-edge distances are indicated by numbers in the parentheses.bAxial amino acid ligands of the heme cofactors.cHeme superposition betweenE. coli,G. th, andMsm.dThe superimposed hemedsites fromMsmandE. coli. Data acquisition was achieved by using serialEM [39] . Images were collected with 40 frames and a total dose of 60 e − /Å 2 . The defocus range was set to 1.2–1.8 μm. For cytochrome bd–aurachin D complex, images were recorded using an FEI Titan Krios electron microscopy operating at 300 kV with a Gatan K2 detector at a magnification of ×165,000 with an energy filter, corresponding to a pixel size of 0.82 Å/pixel. Images were collected with 40 frames and a total dose of 60 e − /Å 2 with a defocus range between 1.2 and 1.8 μm. Image processing Dose-fractioned images were motion-corrected and dose-weighted by MotionCor2 software [40] . CTF estimation was performed by cryoSPARC [41] . 1,578,284 particles were automatically picked and extracted with a box size of 256 pixels [41] . 2D classification and 3D classification and refinement were all performed in cryoSPARC [41] . 50,000 particles were used to generate three classes in ab-initio reconstruction. The classes were used as templates for heterogeneous refinement with all selected particles. After a few rounds of heterorefinement, 270,938 particles converged into one class with a 3.4 Å initial map. These particles were used to perform a homogeneous refinement and local refinement to obtain a final resolution of 2.79 Å. Model building and refinement The final map was sharpened automatically using a B -factor of 121.3 Å 2 in cryoSPARC. The atomic model was manually built in Coot [42] (version 0.8.9.1) using the crystal structure of G.th cytochrome bd (PDB: 5doq) [19] as a template. Real-space refinement and validation of the final model were performed in Phenix (version 1.14) [43] . The local resolution map was calculated with ResMap [44] . All reported resolutions were based on the gold-standard FSC 0.143 criteria [45] . 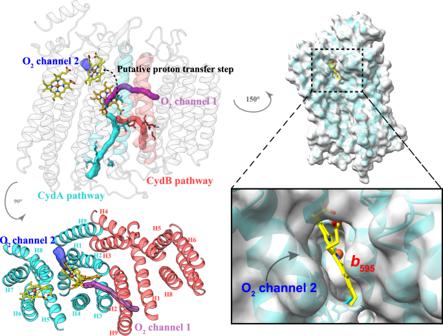Fig. 4: Proton/gaseous substrate channels in theMsm bdoxidase. Subunits CydA/B are shown in cartoon representation. The putative dioxygen and proton channels are labeled. The heme groups are shown as stick models. The proton transfer step from hemeb595to hemedis identified by a black dashed path. 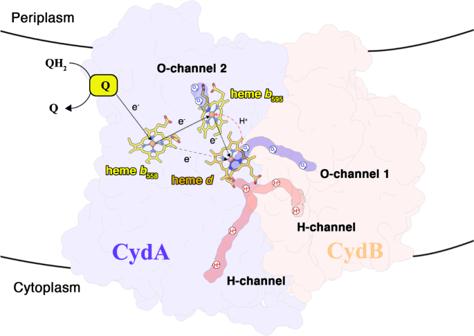Fig. 5: A schematic diagram showing the electron/proton transfer pathway inMsm bdoxidase and the relevant oxygen entry pathway. The heme groups are shown as in stick models. The putative dioxygen and proton channels are labeled. Electron transfer directions are shown in black arrows. FSC work and FSC test were conducted to check for over fitting [46] . All figures were created using UCSF Chimera [47] or PyMOL [48] . Reporting summary Further information on research design is available in the Nature Research Reporting Summary linked to this article.